Band structure engineering in (Bi1−xSbx)2Te3ternary topological insulators Topological insulators (TIs) are quantum materials with insulating bulk and topologically protected metallic surfaces with Dirac-like band structure. The most challenging problem faced by current investigations of these materials is to establish the existence of significant bulk conduction. Here we show how the band structure of topological insulators can be engineered by molecular beam epitaxy growth of (Bi 1− x Sb x ) 2 Te 3 ternary compounds. The topological surface states are shown to exist over the entire composition range of (Bi 1− x Sb x ) 2 Te 3 , indicating the robustness of bulk Z 2 topology. Most remarkably, the band engineering leads to ideal TIs with truly insulating bulk and tunable surface states across the Dirac point that behaves like one-quarter of graphene. This work demonstrates a new route to achieving intrinsic quantum transport of the topological surface states and designing conceptually new topologically insulating devices based on well-established semiconductor technology. The topological surface states of three-dimensional topological insulators (TIs) possess a single spin-polarized Dirac cone originated from strong spin–orbit coupling [1] , [2] , [3] . The unique surface states are expected to host exotic topological quantum effects [4] , [5] , [6] , and find applications in spintronics and quantum computation. The experimental realization of these ideas requires fabrication of versatile devices based on bulk-insulating TIs with tunable surface states. However, the currently available TI materials exemplified by Bi 2 Se 3 and Bi 2 Te 3 (ref. 7 ) always show conductive bulk states due to the defect-induced charge carriers. Tuning the band structure of the TIs to eliminate the bulk states is one of the most urgent tasks in the field, but the problem remains unsolved despite extensive efforts involving nanostructuring [8] , chemical doping [9] , [10] , [11] , [12] , [13] , [14] , [15] and electrical gating [16] , [17] , [18] , [19] . Energy band engineering in conventional semiconductor is a powerful approach for tailoring the electronic structure of materials [20] . A notable example is the isostructural isovalent alloy of the III–V semiconductors Al x Ga 1− x as grown on GaAs by molecular beam epitaxy (MBE), in which the energy gap can be tuned continuously by the mixing ratio of AlAs and GaAs. Such energy band tuning has been essential for heterostructures, which were later used for discovery of fractional quantum Hall effect and invention of high-speed electronics. Inspired by this idea, we conceived a new route for engineering the band structure of TIs by fabricating alloys of Bi 2 Te 3 and Sb 2 Te 3 . Both TIs are V–VI compounds with the same crystal structure and close lattice constants [7] , making it ideal to form (Bi 1− x Sb x ) 2 Te 3 ternary compounds with arbitrary mixing ratio and negligible strain ( Fig. 1a ). The potential advantages of mixing the two TIs can be anticipated from their complementary electronic properties. 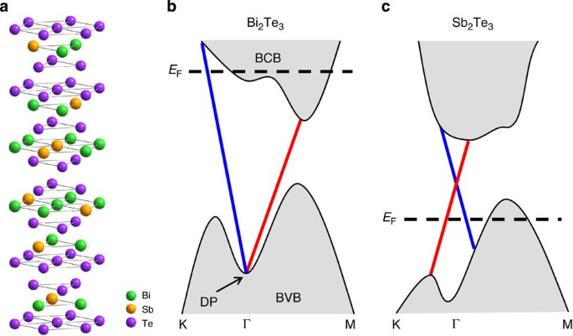Figure 1: The schematic crystal and electronic structures of the (Bi1−xSbx)2Te3compounds. (a) The tetradymite-type crystal structure of (Bi1−xSbx)2Te3where the Bi atoms are partially substituted by Sb. (b) The schematic electronic band structure of pure Bi2Te3and (c) pure Sb2Te3based on theoretical calculations7and ARPES experiments10,21. Figure 1b illustrates the band structure of pure Bi 2 Te 3 (refs 7 , 10 , 21 ), which reveals two major drawbacks of the surface Dirac band in Bi 2 Te 3 . First, the Dirac point (DP) is buried in the bulk valence band (BVB), hence, cannot be accessed by transport experiment and, more seriously, the Fermi level ( E F ) lies in the bulk conduction band (BCB) due to the electron-type bulk carriers induced by Te vacancies. On the other hand, the band structure of pure Sb 2 Te 3 (refs 7 , 21 ), is drastically different. As shown schematically in Figure 1c , here the DP lies within the bulk gap and the E F lies in the BVB due to the hole-type bulk carriers induced by Sb–Te anti-site defects. Intuitively, by mixing the two compounds one can simultaneously achieve charge compensation and tune the position of the DP, which may lead eventually to an ideal TI with exposed DP and insulating bulk. Figure 1: The schematic crystal and electronic structures of the (Bi 1− x Sb x ) 2 Te 3 compounds. ( a ) The tetradymite-type crystal structure of (Bi 1− x Sb x ) 2 Te 3 where the Bi atoms are partially substituted by Sb. ( b ) The schematic electronic band structure of pure Bi 2 Te 3 and ( c ) pure Sb 2 Te 3 based on theoretical calculations [7] and ARPES experiments [10] , [21] . Full size image Here we report the band structure engineering in TIs by fabricating alloys of Bi 2 Te 3 and Sb 2 Te 3 using state-of-the-art MBE. Transport and angle-resolved photoemission spectroscopy (ARPES) measurements show that the band engineering technique allows us to achieve ideal TIs with truly insulating bulk. The surface states can be tuned systematically across the DP and the transport properties are consistent with that of a single spin-polarized Dirac cone. Sample structure During the MBE growth of the (Bi 1− x Sb x ) 2 Te 3 films, the growth rate is calibrated by a real-time reflection high-energy-electron diffraction intensity oscillation measured on the (00) diffraction. Supplementary Figure S1 shows a typical 1×1 reflection high-energy-electron diffraction pattern taken on a (Bi 1− x Sb x ) 2 Te 3 film with five quintuple layers (QLs) thickness. The sharpness of the feature provides a clear evidence for the high quality of the sample. The five QL thickness is used for all (Bi 1− x Sb x ) 2 Te 3 films studied in this work because in this ultrathin regime the surface states dominate charge transport, and meanwhile the films are thick enough that the top and bottom surfaces are completely decoupled. Further discussion about the film thickness issue can be found in the Supplementary Information . Electronic structure The electronic structures of the (Bi 1− x Sb x ) 2 Te 3 films are measured by ARPES on a sample setup as illustrated in Supplementary Figure S2 . 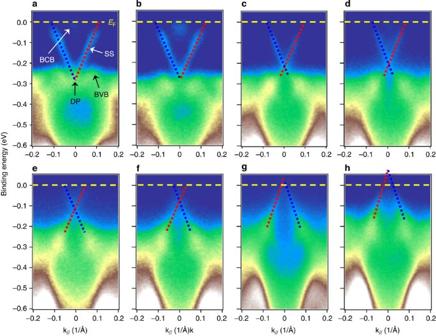Figure 2: ARPES results on the five QL (Bi1−xSbx)2Te3films measured along the K-Γ-K direction. From (a) to (h) the measured band structures of (Bi1−xSbx)2Te3films withx=0, 0.25, 0.62, 0.75, 0.88, 0.94, 0.96 and 1.0, respectively. The Dirac-like topological surface states exist in all films. The yellow dashed line indicates the position of the Fermi level (EF). The blue and red dashed lines indicate the Dirac surface states with opposite spin polarities and they intersect at the DP. The ARPES band maps of eight (Bi 1− x Sb x ) 2 Te 3 films with 0≤ x ≤1 are shown in Figure 2a to h . The pure Bi 2 Te 3 film shows well-defined surface states with massless Dirac-like dispersion ( Fig. 2a ), similar to that of the cleaved Bi 2 Te 3 crystal [10] . With the addition of Sb, the Dirac-like topological surface states can be clearly observed in all (Bi 1− x Sb x ) 2 Te 3 films from x =0 to 1, whereas the Dirac cone geometry changes systematically. With increasing x , the slope of the Dirac line shape becomes steeper, indicating an increase of the Dirac fermion velocity v D defined by the linear dispersion ɛ = v D ·k near the DP. Meanwhile, the E F moves downwards from the BCB, indicating the reduction of the electron-type bulk carriers. Moreover, the DP moves upwards relative to the BVB due to the increasing weight of the Sb 2 Te 3 band structure. When the Sb content is increased to x =0.88 ( Fig. 2e ), both the DP and E F lie within the bulk energy gap. The system is now an ideal TI with a truly insulating bulk and a nearly symmetric surface Dirac cone with exposed DP. Notably, when x increases from x =0.94 ( Fig. 2f ) to 0.96 ( Fig. 2(g) , E F moves from above the DP to below it, indicating a crossover from electron- to hole-type Dirac fermion gas. The charge neutrality point (CNP) where E F meets DP can thus be identified to be located between x =0.94 and 0.96. Figure 2: ARPES results on the five QL (Bi 1− x Sb x ) 2 Te 3 films measured along the K-Γ-K direction. From ( a ) to ( h ) the measured band structures of (Bi 1− x Sb x ) 2 Te 3 films with x =0, 0.25, 0.62, 0.75, 0.88, 0.94, 0.96 and 1.0, respectively. The Dirac-like topological surface states exist in all films. The yellow dashed line indicates the position of the Fermi level ( E F ). The blue and red dashed lines indicate the Dirac surface states with opposite spin polarities and they intersect at the DP. Full size image It is quite remarkable that the topological surface states exist in the entire composition range of (Bi 1− x Sb x ) 2 Te 3 , which implies that the nontrivial Z 2 topology of the bulk band is very robust against alloying. This is in contrast to the Bi 1− x Sb x alloy, the first discovered three-dimensional TI in which the topological surface states only exist within a narrow composition range near x =0.10 (refs 22 , 23 ). 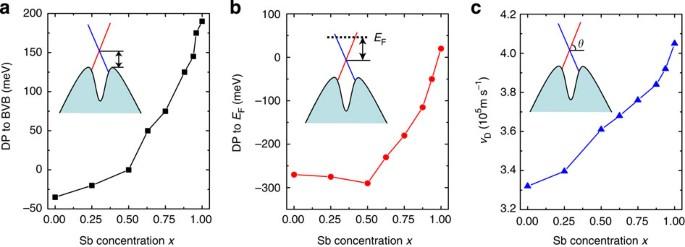Figure 3: Evolution of the surface band characteristics withxobtained from the ARPES data in (Bi1−xSbx)2Te3. (a) Relative position (or energy difference) between the DP and the top of BVB near the Γ point. (b) Relative position between the DP and theEF. (c) The Dirac fermion velocityvD(vD~tanθ) extracted from the linear dispersion near the DP. All three quantities evolve smoothly from that of pure Bi2Te3(x=0) to pure Sb2Te3(x=1). Figure 3a to c summarizes the characteristics of the surface Dirac band in the (Bi 1− x Sb x ) 2 Te 3 compounds, which are extracted following the procedure presented in the Supplementary Information and illustrated in Supplementary Figures S3 and S4 . The position of the DP rises continuously from below the top of BVB near the Γ point at x =0 to way above that at x =1 ( Fig. 3a ). This is accompanied by a drastic change of the relative position of E F and DP ( Fig. 3b ), which determines the type and density of Dirac fermions. Furthermore, v D increases from 3.3×10 5 m s −1 at x =0 to 4.1×10 5 m s −1 at x =1 ( Fig. 3c ). As the three defining properties of the Dirac cone are systematically varied between that of pure Bi 2 Te 3 and Sb 2 Te 3 , the (Bi 1− x Sb x ) 2 Te 3 ternary compounds are effectively a series of new TIs. The bulk electronic structures, including the geometry of BCB and BVB as well as the energy gap between them, are also expected to change with x . They are of interests in their own rights, but will not be the main focus of the current work. Figure 3: Evolution of the surface band characteristics with x obtained from the ARPES data in (Bi 1− x Sb x ) 2 Te 3 . ( a ) Relative position (or energy difference) between the DP and the top of BVB near the Γ point. ( b ) Relative position between the DP and the E F . ( c ) The Dirac fermion velocity v D ( v D ~tanθ) extracted from the linear dispersion near the DP. All three quantities evolve smoothly from that of pure Bi 2 Te 3 ( x =0) to pure Sb 2 Te 3 ( x =1). Full size image Transport properties The systematic Dirac band evolution also manifests itself in the transport properties. 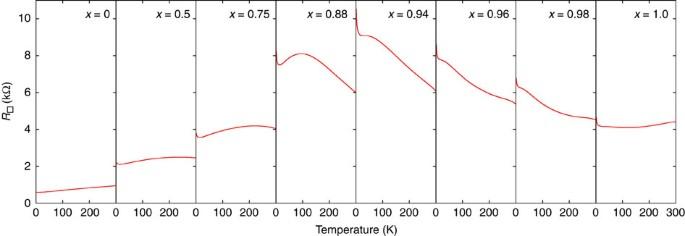Figure 4: Two-dimensional sheet resistance (R□) versus temperature (T) for eight five QL (Bi1−xSbx)2Te3films. R□value keeps rising and the insulating tendency becomes stronger with increasing Sb content fromx=0 to 0.94 due to the reduction of electron-type carriers. Fromx=0.96 to 1 the trend is reversed, that is,R□value decreases and the insulating tendency becomes weaker with increasing Sb content due to the increasing density of hole-type carriers. Figure 4 displays the variation of two-dimensional sheet resistance ( R □ ) with temperature ( T ) for eight QL (five) (Bi 1− x Sb x ) 2 Te 3 films with 0≤ x ≤1. In pure Bi 2 Te 3 the resistance shows metallic behaviour at high T and becomes weakly insulating at very low T . With increasing x , the R □ value keeps rising and the insulating tendency becomes stronger, reflecting the depletion of electron-type bulk carriers and surface Dirac fermions. At x =0.94 when E F lies just above DP, the resistance reaches the maximum value and shows insulating behaviour over the whole T range. With further increase of Sb content from x =0.96 to 1, the resistance decreases systematically because now E F passes DP and more hole-type carriers start to populate the surface Dirac band. The high T metallic behaviour is recovered in pure Sb 2 Te 3 when the hole-type carrier density becomes sufficiently high. Figure 4: Two-dimensional sheet resistance ( R □ ) versus temperature ( T ) for eight five QL (Bi 1− x Sb x ) 2 Te 3 films. R □ value keeps rising and the insulating tendency becomes stronger with increasing Sb content from x =0 to 0.94 due to the reduction of electron-type carriers. From x =0.96 to 1 the trend is reversed, that is, R □ value decreases and the insulating tendency becomes weaker with increasing Sb content due to the increasing density of hole-type carriers. 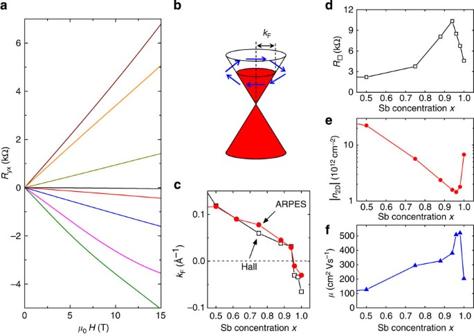Figure 5: The Hall effect and summary of the transport results. (a) The field dependence of the Hall resistanceRyxfor the eight (Bi1−xSbx)2Te3films measured atT=1.5 K. From top to bottom, the curves are the Hall traces of (Bi1−xSbx)2Te3films withx=0.96, 0.98, 1.0, 0, 0.50, 0.75, 0.88 and 0.94, respectively. The evolution of the Hall effect reveals the depletion of electron-type carriers (fromx=0 to 0.94), the reversal of carrier type (fromx=0.94 to 0.96), and the increase of hole-type carrier density (fromx=0.96 to 1.0). (b) Schematic sketch of an isotropic circular Dirac cone where the Fermi wavevectorskFis marked. The blue arrows indicate the helical spin texture. (c) ThekFof the Dirac cone derived from the Hall effect (black open squares) agree well with that directly measured by ARPES (red solid circles) if we assume a single spin-polarized Dirac cone on each surface. ThekFis defined to be negative for hole-type Dirac fermions. The sheet resistanceR□(d), the carrier density |n2D| (e) and the mobilityìof the Dirac fermions (f) measured atT=1.5 K all show “V”-shapedxdependence near the CNP. Full size image Figure 5a displays the variation of the Hall resistance ( R yx ) with magnetic field ( H ) measured on the five QL (Bi 1− x Sb x ) 2 Te 3 films at T =1.5 K. For films with x ≤0.94, the R yx value is always negative, indicating the existence of electron-type carriers. The weak-field slope of the Hall curves, or the Hall coefficient R H , increases systematically with x in this regime. As the two-dimensional carrier density n 2D can be derived from R H as n 2D =1/ eR H ( e is the elementary charge), this trend confirms the decrease of electron-type carrier density with Sb doping. As x increases slightly from 0.94 to 0.96, the Hall curve suddenly jumps to the positive side with a very large slope, which indicates the reversal to hole-type Dirac fermions with a small carrier density. At even higher x , the slope of the positive curves decreases systematically due to the increase of hole-type carrier density. Figure 5: The Hall effect and summary of the transport results. ( a ) The field dependence of the Hall resistance R yx for the eight (Bi 1− x Sb x ) 2 Te 3 films measured at T =1.5 K. From top to bottom, the curves are the Hall traces of (Bi 1− x Sb x ) 2 Te 3 films with x =0.96, 0.98, 1.0, 0, 0.50, 0.75, 0.88 and 0.94, respectively. The evolution of the Hall effect reveals the depletion of electron-type carriers (from x =0 to 0.94), the reversal of carrier type (from x =0.94 to 0.96), and the increase of hole-type carrier density (from x =0.96 to 1.0). ( b ) Schematic sketch of an isotropic circular Dirac cone where the Fermi wavevectors k F is marked. The blue arrows indicate the helical spin texture. ( c ) The k F of the Dirac cone derived from the Hall effect (black open squares) agree well with that directly measured by ARPES (red solid circles) if we assume a single spin-polarized Dirac cone on each surface. The k F is defined to be negative for hole-type Dirac fermions. The sheet resistance R □ ( d ), the carrier density | n 2D | ( e ) and the mobility ì of the Dirac fermions ( f ) measured at T =1.5 K all show “V”-shaped x dependence near the CNP. Full size image The evolution of the Hall effect is totally consistent with the surface band structure revealed by ARPES in Figure 2 . To make a more quantitative comparison between the two experiments, we use the n 2D derived from the Hall effect to estimate the Fermi wavevector k F of the surface Dirac band. By assuming zero bulk contribution and an isotropic circular Dirac cone structure ( Fig. 5b ), k F can be expressed as Here D is the degeneracy of the Dirac fermion and is the carrier density per surface if we assume that the top and bottom surfaces are equivalent. Figure 5c shows that when we choose D =1, the k F values derived from the Hall effect match very well with that directly measured by ARPES. This remarkable agreement suggests that the transport properties of the TI surfaces are consistent with that of a single spin-polarized Dirac cone, or a quarter of graphene, as expected by theory. Figure 5d to f summarizes the evolution of the low T transport properties with Sb content x . The resistance value shows a maximum at x =0.94 with R □ > 10 kΩ and decreases systematically on both sides. Correspondingly, the carrier density | n 2D | reaches a minimum at x =0.96 with | n 2D |=1.4×10 12 cm −2 and increases on both sides. Using the measured R □ and | n 2D |, the mobility μ of the Dirac fermions can be estimated by using the Drude formula σ 2D =| n 2D | eμ , where σ 2D =1/ R □ . As a function of x the mobility also peaks near the CNP and decreases rapidly on both sides. The 'V'-shaped dependence of the transport properties on the Sb content x clearly demonstrates the systematic tuning of the surface band structure across the CNP. The good agreement with ARPES suggests that the transport results are consistent with the properties of the surface Dirac fermions without bulk contribution. Moreover, the alloying allows us to approach the close vicinity of the CNP, which gives a very low | n 2D | in the order of 1×10 12 cm −2 . The (Bi 1− x Sb x ) 2 Te 3 compounds thus represent an ideal TI system to reach the extreme quantum regime because now a strong magnetic field can squeeze the Dirac fermions to the lowest few Landau levels. Indeed, the Hall resistance of the x =0.96 film shown in Figure 5a is close to 7 kΩ at 15 T, which is a significant fraction of the quantum resistance. Future transport measurements on (Bi 1− x Sb x ) 2 Te 3 films with higher mobility to even stronger magnetic field hold great promises for uncovering the unconventional quantum Hall effect of the topological surface states [24] , [25] . The band structure engineering offers many enticing opportunities for designing conceptually new experimental or device schemes based on the TIs. For example, we can apply the idea of compositionally graded doping (CGD) in conventional semiconductor devices [20] to the TIs to achieve spatially variable Dirac cone structures. 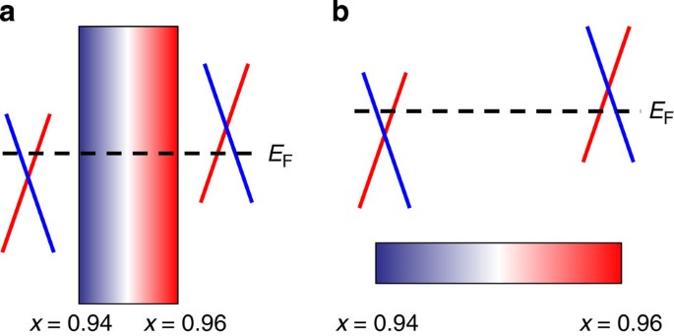Figure 6: Schematic device structures of spatially variable Dirac bands grown by CGD of (Bi1−xSbx)2Te3films. Vertical CGD TIs (a) is an ideal system for studying the topological exciton condensation and electrical control of spin current. Horizontal CGD TIs (b) can be used to fabricate a topologicalp–njunction. Figure 6a illustrates the schematic of vertical CGD TIs, in which the top and bottom surfaces have opposite types of Dirac fermions and can be used for studying the proposed topological exciton condensation [26] . The spatial asymmetry of the surface Dirac bands can also be used to realize the electrical control of spin current by using the spin-momentum locking in the topological surfaces for spintronic applications [27] . Figure 6b illustrates the schematic of horizontal CGD TIs, by which a topological p–n junction between hole- and electron-type TIs can be fabricated. Figure 6: Schematic device structures of spatially variable Dirac bands grown by CGD of (Bi 1− x Sb x ) 2 Te 3 films. Vertical CGD TIs ( a ) is an ideal system for studying the topological exciton condensation and electrical control of spin current. Horizontal CGD TIs ( b ) can be used to fabricate a topological p–n junction. Full size image MBE sample growth The MBE growth of TI films on insulating substrate has been reported before by the same group [28] . The (Bi 1− x Sb x ) 2 Te 3 films studied here are grown on sapphire (0001) in an ultra-high vacuum MBE-ARPES-STM combined system with a base pressure of 1×10 10 Torr. Before sample growth, the sapphire substrates are first degassed at 650 °C for 90 min and then heated at 850 °C for 30 min. High-purity Bi (99.9999%), Sb (99.9999%) and Te (99.999%) are evaporated from standard Knudsen cells. To reduce Te vacancies, the growth is kept in Te-rich condition with the substrate temperature at 180 °C. The Bi:Sb ratio is controlled by the temperatures of the Bi and Sb Knudsen cells. The x value in the (Bi 1− x Sb x ) 2 Te 3 film is determined through two independent methods, as discussed in detail in Supplementary Information . ARPES measurements The in situ ARPES measurements are carried out at room temperature by using a Scienta SES2002 electron energy analyser. A Helium discharge lamp with a photon energy of hν =21.218 eV is used as the photon source. The energy resolution of the electron energy analyser is set at 15 meV. All the spectra shown in the paper are taken along the K-Γ-K direction. To avoid sample charging during ARPES measurements due to the insulating sapphire substrate, a 300-nm-thick titanium film is deposited at both ends of the substrate, which is connected to the sample holder. The sample is grounded through these contacts once a continuous film is formed. The sample setup for the ARPES measurements is illustrated schematically in the Supplementary Figure S2 . Transport measurements The transport measurements are performed ex situ on the five QL (Bi 1− x Sb x ) 2 Te 3 films grown on sapphire (0001) substrate. To avoid possible contamination of the TI films, a 20-nm thick amorphous Te capping layer is deposited on top of the films before we take them out of the ultra-high vaccum growth chamber for transport measurements. The Hall effect and resistance are measured using standard ac lock-in method with the current flowing in the film plane and the magnetic field applied perpendicular to the plane. The schematic device setup for the transport measurements is shown in Supplementary Figure S5 . The 20-nm amorphous Te capping layer causes no significant change of the TI surface electronic structure and makes negligible contribution to the total transport signal, as shown in Supplementary Figure S6 and discussed in the Supplementary Information . How to cite this article: Zhang, J. et al . Band structure engineering in (Bi 1− x Sb x ) 2 Te 3 ternary topological insulators. Nat. Commun. 2:574 doi: 10.1038/ncomms1588 (2011).